Total syntheses of shizukaols A and E Shizukaols possess a common heptacyclic framework containing more than ten contiguous stereocenters and potential biological activities. Here we report that the total syntheses of shizukaols A ( 1 ) and E ( 2 ), two lindenane-type dimers from the Chloranthaceae family, are achieved via a modified biomimetic Diels–Alder reaction. The common crucial biomimetic diene 23 and ethylene species ( 6 , 17 ) are obtained through either a highly Z -selective olefination of α-siloxy ketone with ynolate anions or an intramolecular Horner–Wadsworth–Emmons olefination from commercially available Wieland–Miescher ketone ( 7 ). This synthetic approach here opens up practical avenues for the total syntheses of the intriguing Chloranthaceae family members, as well as the understanding of their relevant biological action in nature. In 1990, shizukaol A ( 1 ) (Fig. 1 ) was isolated from Chloranthus japonicus [1] , [2] as the first dimeric lindenane-type sesquiterpenoid. Subsequently, shizukaol E ( 2 ) (Fig. 1 ) was successively isolated from Chloranthus japonicus in 1995 [3] , [4] . To date, >110 congeners with a similar polycyclic core have been identified from the Chloranthaceae family [5] , [6] , [7] . These molecules possess a common heptacyclic framework containing >10 contiguous stereocenters. Noteworthy is that shizukaol E ( 2 ) showed potential anti-HIV-1 replication activities and significant inhibition effects against the currently most popular NNRTI-resistant HIV-1, together with the inhibitory activities on HCV replication, making it attractive as a potential therapy against the co-infection of HIV-1 and HCV [8] . In addition, most of these dimeric lindenane-type molecules show impressive bioactivities, such as remarkable cytotoxicity [9] , inhibition of the delayed rectifier K + current [10] , [11] , and antimalarial activities [12] . Therefore, the promising bioactivities and synthetic challenges arising from these unprecedented molecules have initiated a significant interest to synthetic chemists [13] , [14] , [15] , [16] , [17] , [18] , [19] , [20] , [21] , [22] , [23] , [24] , [25] , [26] , [27] , [28] , [29] , [30] . However, only one total synthesis of two dimeric members [30] and a number of relevant synthetic studies [13] , [14] , [15] , [16] , [17] , [18] , [19] , [20] , [21] , [22] , [23] , [24] , [25] , [26] , [27] , [28] , [29] have been achieved. In 2017, Liu and coworkers reported the first total syntheses of the dimeric shizukaol D ( 3 ) and sarcandrolide J ( 4 ) [30] through a cascade protocol featuring furan formation/alkene isomerization/Diels–Alder reaction. As shown in Fig. 2 , the pyrolysis of shizukaol A ( 1 ) in a sealed tube resulted in a retro Diels–Alder fragmentation of the linking six-membered ring to furnish two products: the relatively unstable diene 5 and the previously known chloranthalactone A ( 6 ) [1] , [2] . This led to a biogenetic hypothesis for the lindenane dimeric family in which enzymatic endo -Diels–Alder reaction of two lindenane-type components (such as 5 and 6 ) forms a common linking six-membered ring. Based on this hypothesis, we have illustrated a practical strategy for constructing the heptacyclic framework of the Chloranthaceae family via an endo- Diels–Alder reaction as the pivotal step, as shown in Fig. 2 [28] , [29] . Encouraged by our preliminary results of endo- Diels–Alder reaction [28] , [29] , herein we accomplished the total syntheses of two members of this dimeric family, shizukaols A ( 1 ) and E ( 2 ), through mimicking a biosynthetic approach. Fig. 1 Structures of dimeric lindenane-type representives. Shizukaol family possesses a common heptacyclic framework with >10 contiguous stereocenters Full size image Fig. 2 Pyrolysis of shizukaol A. Shizukaol A was pyrolysized to afford relatively unstable diene 5 and known chloranthalactone A ( 6 ) via a retro Diels–Alder fragmentation of the linking six-membered ring in a sealed tube Full size image Retrosynthetic analysis Inspired by our preliminary investigations [28] , [29] on endo- Diels–Alder reaction to generate heptacyclic framework of the Chloranthaceae family, we considered to design more suitable precusors, being at least biogenetically much closer to components 5 and 6 for further transformation. Inspection of the structures of shizukaols A ( 1 ) and E ( 2 ) reveals a linking six-membered ring and a hydroxyl ketoester moiety to be the common structural features of many dimeric lindenane-type molecules. In consideration of the likely instability of 5 , as well as the long synthetic steps in the conversion of our preliminary [4+2] cycloaddition products to shizukaol A ( 1 ), we reason that the synthesis of a crucial heptacyclic core with suitable functional groups for subsequent conversions to naturally occurring shizukaols A ( 1 ) and E ( 2 ) should be a more practical approach. Moreover, our preliminary investigation proved that the late-stage conversion of the epoxy unit in 9 (Fig. 3 ) to the hydroxyl ketoester unit of shizukaols A ( 1 ) and E ( 2 ), a common framework of the dimeric family members, is a more step-economic strategy for total syntheses. In addition, the epoxide moiety in triene 9 is expected to prevent a further [4+2] cycloaddition of relevant alkenyl unit. Therefore, on basis of these considerations and the aforementioned biogenetic hypothesis, we think that the critical step for the construction of skeleton relevant to that of shizukaols A ( 1 ) and E ( 2 ) would then be the expedient and pragmatic conversion of readily accessible precursor 10 and biomimetic epoxide 9 into the endo- Diels–Alder reaction product 11 via the relevant transition state. Upon endo- Diels–Alder reaction of 9 and 10 , epoxy compound 11 could readily be obtained which then undergoes a biomimetic transformation of epoxy unit to the common hydroxyl ketoester species of the shizukaol family, eventually achieving shizukaols A ( 1 ) and E ( 2 ). Fig. 3 Retrosynthetic analysis toward shizukaols A and E. This proposed protocol is featuring with a modified biomimetic approach involving an endo- Diels–Alder reaction and biomimetic transformation Full size image Total syntheses of shizukaols A and E Based on the aforementioned synthetic strategy, we then commenced the synthesis of ethylene 17 from known compound 12 (Fig. 4 ) [28] , [29] , which was obtained through the sequence of classical Mitsunobu reaction [31] , [32] , nickel-mediated reduction [33] , [34] , and modified Julia–Kocienski olefination (see Supporting Information for details) [35] . Compound 12 was then treated with 9-BBN to form an inseparable mixture of diastereoisomers in a ratio of 8:1 ( α / β ). Deprotection with FeCl 3 •SiO 2 led to alcohol 13 with an α-hydroxymethyl group as the major product. It is noteworthy that Zhao and coworkers reported the synthesis of the single stereoisomer of 13 with β-hydroxymethyl group under a similar hydroboration condition [19] . Therefore, in order to further identify the stereochemistry, protection of hydroxyl group in 13 with p- nitrobenzoyl group provided compound 13a in a quantitative yield. After many trials, compound 13a gave finally satisfactory single crystals from CH 2 Cl 2 , whose X-ray diffraction study convincingly showed an α-hydroxymethyl group in 13a to be consistent with its relevant orientation in shizukaol E ( 2 ). The stereoselectivity of this hydroboration is presumably caused by the presence of 1,3- syn -diaxial repulsion in alkene 12 . Subsequent protection of the primary alcohol with a TBS group gave ketone 14 , which reacted with Bredereck’s reagent and singlet oxygen successfully to form dione 15 in 77% yield [36] , [37] . The resulting dione 15 underwent Yamaguchi esterification [38] with commercially available 2-(diethoxyphosphoryl)propanoic acid ( 15a) and 2,4,6-trichlorobenzoyl chloride ( 15b ) to furnish an easily separable mixture of 16 and its regioisomer 16a in 59% and 25% yields, respectively. The undesired regioisomer 16a could be recycled into dione 15 in 81% yield in the presence of Na 2 CO 3 . Then, treatment of 16 with NaH in THF led to the desired ethylene 17 in 77% yield. Fig. 4 Synthesis of ethylene 17. 9-BBN 9-borabicyclo[3.3.1]nonane, TBS tert-butyldimethylsilyl, DMAP 4-dimethylaminopyridine, DMP Dess–Martin periodinane Full size image With ethylene 17 in hand, we turned our attention to the synthesis of diene 23 from known enone 18 [28] , [29] . As shown in Fig. 5 , regio- and stereoselective dihydroxylation of enone 18 in the presence of a catalytic amount of OsO 4 and one equivalent of NMO afforded exclusively the corresponding diol from the less-hindered α-face. Upon regioselective protection of the less sterically hindered secondary alcohol with a TBS group, α-siloxy ketone 19 was furnished in 70% yield. The regioselectivity of silylation could be ascribed to the steric hindrance of the angular methyl and the bulky silyl group. Next, treatment of α-siloxy ketone 19 with freshly prepared ynolate 19a led to a highly Z -selective olefination of 19 under a mild condition [39] , [40] , [41] . As a result, butenolide 20 was smoothly generated via a spontaneous silyl migration and lactonization. Moreover, the stereochemistry of 20 was confirmed through an X-ray crystallographic analysis of a single crystal of butenolide 20 grown from CH 2 Cl 2 . Lactone 20 was then allowed to undergo elimination of OTBS with DBU to generate 21 in 80% yield, which increased to 93% yield after recovery of 20 . As shown in Fig. 3 , we predicted that β-epoxide would facilitate subsequent transformation. Lamentably, we failed to form directly the β-epoxide from alkene 21 after considerable testing of epoxidation protocols. Similarly, we failed to convert the α-epoxide of compound 22 into β-epoxide after extensive efforts. We therefore planned to reverse its relevant stereochemistry at a later stage. Epoxidation of 21 with m -CPBA led exclusively to α-epoxide 22 . Then, dehydration of 22 with Martin sulfurane smoothly gave rise to triene 23 [42] , [43] , which was very unstable and easy to dimerize in its neat form or undiluted solution. Fortunately, diene 23 was relatively stable when diluted in toluene or xylene and stored at −20 °C for immediate use without obvious dimerization or polymerization. Fig. 5 Synthesis of diene 23 . NMO N -methylmorpholine N -oxide, TBS tert -butyldimethylsilyl, DMAP 4-dimethylaminopyridine, DBU 1,8-diazabicyclo[5.4.0]undec-7-ene, and m -CPBA meta -chloroperbenzoic acid Full size image Next, we investigated the possibility of an endo -Diels–Alder reaction between electron-deficient electrophilic diene 23 and electron-rich C8′–C9′ double bond of nucleophilic ethylene 17 [44] , [45] , [46] . As shown in Fig. 6 , treatment of compounds 17 and 23 with butylated hydroxytoluene (BHT) at 160 °C in xylene successfully led to the endo- Diels–Alder reaction cycloadduct 24 as a single detectable isomer. Noteworthy, the homo-dimerization product of diene 23 was observed as the major by-product of this Diels–Alder reaction. Therefore, in order to reduce the homo-dimerization of diene 23 , it is essential for endo -Diels–Alder reaction that a high dilute solution of 23 was added into a refluxing dilute solution of 17 very slowly. Then, removal of the silyl group in 24 led to the crucial alcohol 25 in 87% yield as a solid. After many trials, alcohol 25 gave eventually satisfactory single crystals from CH 2 Cl 2 . Its X-ray diffraction study confirmed that alcohol 25 was the desired endo- Diels–Alder reaction product. However, efforts to improve this Diels–Alder reaction using Lewis acid/base catalysts caused decomposition of the sensitive substrates. Therefore, this thermal Diels–Alder reaction appears to be an acceptable approach for generating 24 as a single detectable dimer. With alcohol 25 in hand, it was then allowed to undergo hydrolysis with K 2 CO 3 to generate the corresponding diol, thereby installing the crucial hydroxyl ketoester moiety of the natural product family in a biomimetic transformation. Selective acetylation of the primary alcohol then provided monoacetate 26 in 72% yield in two steps. Next, efforts to invert the secondary α-hydroxyl group in 26 were unsuccessful, probably because the hydroxy group at C9 of 26 was sterically hindered. Even the corresponding mesylate and triflate, which were easily epimerized, did not give positive results when treated with alkaline reagents such as DBU and KNO 2 [47] . Therefore, oxidation of alcohol 26 with Dess–Martin periodinane led to the dione 27 . Treatment of 27 with Zn(BH 4 ) 2 eventually gave the synthetic shizukaol E ( 2 ) with a C9 β-hydroxyl group, together with recyclable compound 26 in 92% yield with an α / β ratio of 2.8:1 (see Supplementary Table 3 ). The synthetic shizukaol E ( 2 ) was fully characterized, and its NMR spectroscopic data are identical to those reported in the literature [3] , [4] . 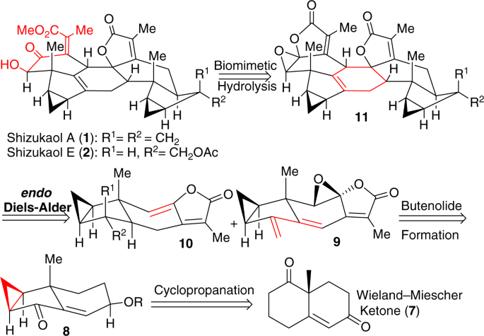Fig. 3 Retrosynthetic analysis toward shizukaols A and E. This proposed protocol is featuring with a modified biomimetic approach involving anendo-Diels–Alder reaction and biomimetic transformation However with the exception of Zn(BH 4 ) 2 , other reductive reagents such as NaBH 4 , L-selectride, etc. resulted in much lower stereoselectivity than that of Zn(BH 4 ) 2 . 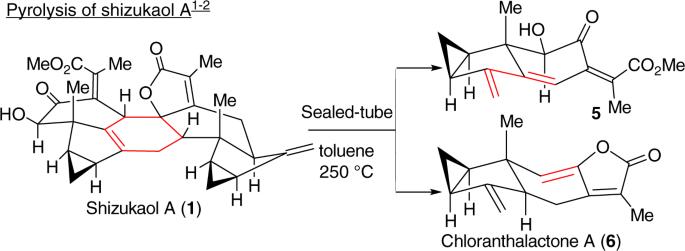Some reducing reagents such as LiAl( t BuO) 3 H even led only to compound 26 with α-selectivity. 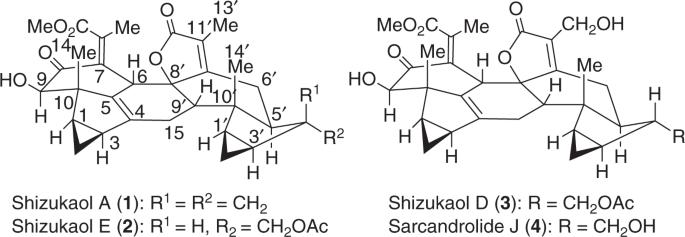Fig. 2 Pyrolysis of shizukaol A. Shizukaol A was pyrolysized to afford relatively unstable diene5and known chloranthalactone A (6) via a retro Diels–Alder fragmentation of the linking six-membered ring in a sealed tube Presumably, the stereoselectivity of this reduction results from coordination between Zn(BH 4 ) 2 and the two carbonyl groups at C8 and C9 in dione 27 . Fig. 1 Structures of dimeric lindenane-type representives. Shizukaol family possesses a common heptacyclic framework with >10 contiguous stereocenters 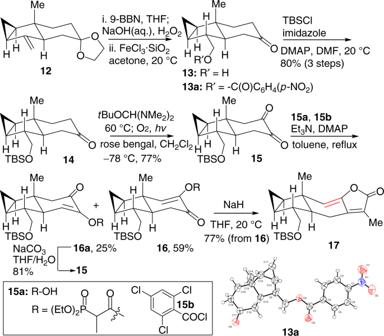Fig. 4 Synthesis of ethylene 17. 9-BBN 9-borabicyclo[3.3.1]nonane, TBS tert-butyldimethylsilyl, DMAP 4-dimethylaminopyridine, DMP Dess–Martin periodinane The relevant DFT calculations of the reduction of dione 27 with Zn(BH 4 ) 2 was performed using Gaussian 09 to understand the observed stereoselectivity (see Supplementary Table 12 and Supplementary Figure 4 ). Fig. 6 Total synthesis of shizukaol E ( 2 ). BHT butylated hydroxytoluene, DMP Dess–Martin periodinane, DMAP 4-dimethylaminopyridine Full size image With the completion of the total synthesis of shizukaol E ( 2 ), we then concerned on the total synthesis of shizukaol A ( 1 ). As shown in Fig. 7 , when ethylene glycol in compound 12 was removed with FeCl 3 •SiO 2 in acetone, the resulting ketone underwent a conversion similar to the transformation of 14 to 15 . Subsequent sun-lamp irradiation afforded exclusively dione 28 in 75% overall yield for two steps. Upon a similar procedure as described above, regioselective Yamaguchi esterification of dione 28 followed by intramolecular Horner–Wadsworth–Emmons olefination [48] finally gave rise to chloranthalactone A ( 6 ) as nucleophilic ethylene for Diels–Alder reaction. During workup and purification process, 6 was partially oxidized to the respective epoxide in air. Then, exposure of 6 and 23 under a thermal condition provided exclusively the desired endo -Diels–Alder cycloadduct 29 . To better understand the observed stereochemical outcome of the endo -Diels–Alder reaction between diene 23 and ethylene species 17 or 6 , we carried out computational studies of diene 23 and ethylene 6 using Gaussian 09 [49] , and the relevant results were consistent with our experimental observations (see Supporting Information for details). Subsequently, a biomimetic hydrolysis with KOH in MeOH gave compound 30 in 72% yield. Oxidation of 30 with Dess–Martin periodinane followed by reduction of dione 31 with Zn(BH 4 ) 2 , eventually achieved shizukaol A ( 1 ) and alcohol 30 in 95% yield with an α / β ratio of 4.6:1. The spectroscopic data of synthetic shizukaol A ( 1 ), including MS, IR, and NMR, are in full agreement with those reported [1] , [2] . Fig. 7 Total synthesis of shizukaol A ( 1 ). DMAP 4-dimethylaminopyridine, BHT butylated hydroxytoluene, DMP Dess–Martin periodinane Full size image In summary, we achieved the first total syntheses of shizukaols A ( 1 ) and E ( 2 ) from commercially available Wieland–Miescher ketone ( 7 ) through mimicking the modified biogenetic pathway in 0.1% overall yield over 24 steps and 0.15% overall yield over 28 steps in the longest linear sequence, respectively. According to the structural features of the shizukaol family, an efficient butenolide formation was developed for the synthesis of the common biomimetic diene 23 and ethylene species ( 6 and 17 ) using either a highly Z -selective olefination of α-siloxy ketone with ynolate anions or an intramolecular Horner–Wadsworth–Emmons olefination. Inspired by the hypothetical biogenetic pathway for the shizukaol family and the pyrolysis results, we proposed and validated a modified biomimetic approach involving an endo- Diels–Alder reaction and biomimetic transformation. This methodology may be practical for the syntheses of other members in the intriguing Chloranthaceae family, as well as other potential lead molecules for understanding of their relevant biological action and biogenetically synthetic protocol in nature. General All reagents and solvents were of reagent grade. Further purification and drying following the guidelines of Perrin and Armarego [50] were used when necessary. Organic solvents were concentrated under reduced pressure on a rotary evaporator in a water bath no more than 40 ℃ unless otherwise specified. Thin-layer chromatography (TLC) was performed on E. Merck silica gel 60 F254 (0.25 mm thickness) coated on aluminum plates. Chromatographic purification of products was performed on Macherey–Nagel–Kieselgel 60 M (230–400 mesh). Visualization of the developed chromatogram was performed by acidic ceric ammonium molybdate and subsequent heating. 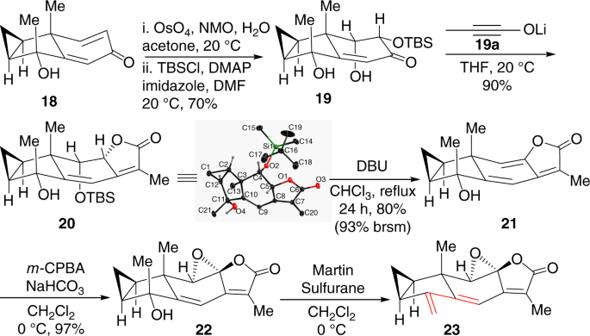Fig. 5 Synthesis of diene23. NMON-methylmorpholineN-oxide, TBStert-butyldimethylsilyl, DMAP 4-dimethylaminopyridine, DBU 1,8-diazabicyclo[5.4.0]undec-7-ene, andm-CPBAmeta-chloroperbenzoic acid Melting points were measured with a Stuart Melting Point Apparatus (SMP40) in Celsius degrees and were uncorrected. 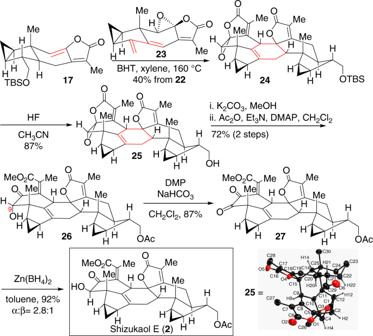Fig. 6 Total synthesis of shizukaol E (2). BHT butylated hydroxytoluene, DMP Dess–Martin periodinane, DMAP 4-dimethylaminopyridine 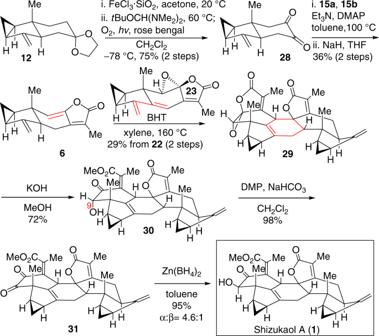Fig. 7 Total synthesis of shizukaol A (1). DMAP 4-dimethylaminopyridine, BHT butylated hydroxytoluene, DMP Dess–Martin periodinane Nuclear magnetic resonance (NMR) spectra were recorded with a Bruker ADVANCE-III NMR spectrometer at 400.13 MHz ( 1 H) or at 100.6 MHz ( 13 C). All NMR measurements were carried out in CDCl 3 and internally referenced to residual solvent signals (referenced at δ 7.26 ppm in 1 H, and δ 77.16 ppm for central line of the triplet in 13 C). Data for 1 H NMR are reported as follows: chemical shift (δ ppm), multiplicity (s = singlet, d = doublet, t = triplet, q = quartet, brs = broad singlet, dd = doublet of doublets, dt = doublet of triplets, td = triplet of doublets, ddd = doublet of doublets of doublets, m = multiplet), integration, coupling constant (Hz), and assignment. Data for 13 C NMR are reported in terms of chemical shift. Mass spectrometry (MS) and high-resolution mass spectrometry (HRMS) were measured on a ThermoFinnigan MAT 95XL. Elemental analyses were carried out by Shanghai Institute of Organic Chemistry, the Chinese Academy of Science, PRC. Selected crystals for X-ray analyses were used for intensity data collection on either a Bruker AXS Kappa Apex II Duo diffractometer or Bruker D8 Venture X-Ray Diffractometer at 173 K using frames of oscillation range 0.3°, with 2° < θ < 28°. Infrared spectra (IR) were recorded on a Nicolet 420 FT-IR spectrometer as thin film on potassium bromide discs.